The nucleosome acidic patch plays a critical role in RNF168-dependent ubiquitination of histone H2A During DNA damage response, the RING E3 ligase RNF168 ubiquitinates nucleosomal H2A at K13–15. Here we show that the ubiquitination reaction is regulated by its substrate. We define a region on the RING domain important for target recognition and identify the H2A/H2B dimer as the minimal substrate to confer lysine specificity to the RNF168 reaction. Importantly, we find an active role for the substrate in the reaction. H2A/H2B dimers and nucleosomes enhance the E3-mediated discharge of ubiquitin from the E2 and redirect the reaction towards the relevant target, in a process that depends on an intact acidic patch. This active contribution of a region distal from the target lysine provides regulation of the specific K13–15 ubiquitination reaction during the complex signalling process at DNA damage sites. Ubiquitin conjugation is a regulatory post-translational modification employed by the cell in a variety of processes [1] . A three-step cascade of E1, E2 and E3 enzymes is required for the reaction and the molecular mechanism of the ubiquitination process varies with the target and the enzymes involved. Target specificity in the ubiquitination reaction is regulated in most cases by the E3 ligases [2] that can mono-, multi- or poly-ubiquitinate their substrates. The vast majority of these proteins function through a structurally conserved RING domain that is able to allosterically activate the E2~ubiquitin complex to release the ubiquitin moiety directly onto the lysine residue of the selected substrate [3] . In some cases, the modification site on the substrate is relatively undefined (for example, on p53, p27 and DDB2) [4] , [5] , [6] . In other cases, E3 ligase reactions are highly specific for a single residue (for example, PCNA, IκB, H2B and H2A) [7] , [8] , [9] , [10] , [11] , [12] , [13] , [14] , [15] , [16] . The difference in the stringency of the site specificity of the E3 reactions highlights the diversity of signals generating from ubiquitination events. Some ubiquitin signals do not require a specific attachment site on the substrate, as they signal primarily through the ubiquitin moieties (for example, K48 chains for proteasomal degradation). However, in those cases where ubiquitination stimulates a specific molecular signal, the choice of target lysine must be restricted, resulting in a highly selective E3 reaction. Examples include the site-specific mono-ubiquitination of PCNA, H2B and H2A, which are recognized by specific interacting proteins, thus providing a selective signalling response [17] , [18] , [19] , [20] , [21] . How RING E3 ligases determine target selection is highly variable. In some classes of RING E3s components outside the RING domain are responsible for target selection. For instance, in the family of Cullin-RING Ligases (CRLs) substrate recognition involves a separate molecule besides the subunit carrying the RING domain [22] . Similarly, for some RING E3s not belonging to the CRL family (for example, CHIP and c-Cbl) [23] , [24] , domains outside the RING motif are required for target recognition. In other cases, the isolated RING domains appear to be sufficient for lysine specificity [13] , [14] , [25] . In these instances, a selective RING/E2~Ub–substrate interaction must occur to orient the ubiquitination machinery to the correct lysine. However, the RING is situated at least 20–30 Å away from the active site cysteine on the E2 enzyme where the C-terminal end of ubiquitin forms a thioester bond, ready to be attacked by the amino group of the target lysine. This implies that a region of the substrate, relatively far from the target lysine, may be involved in the ubiquitination reaction. The molecular mechanism of activation of the E2~Ub complex by the RING domain of E3s has recently been clarified by several studies [26] , [27] , [28] . These show how the RING domain and the ubiquitin-charged E2 form a trimeric complex that positions ubiquitin in a conformation proficient for efficient release onto the substrate lysine. In this orientation, the donor ubiquitin makes contact with the E2 via the I44 hydrophobic patch and a salt bridge via its R42, but also engages interactions with the E3 via residues of the I36 hydrophobic patch [26] , [27] , [28] , [29] , [30] . Stabilization of this state is a largely conserved mechanism among different RING-mediated reactions and mutation of these residues on ubiquitin affects E2 discharge and target modification. However, in this rather detailed mechanistic description of the ubiquitination reaction by RING domains, the role of the target molecule has thus far been poorly defined. Molecular insights on the potential catalytic roles of targets so far have been restricted to ubiquitin itself as a substrate during the formation of specific chain types by E2-conjugating enzymes [29] , [30] . Here we investigate the relative contributions of E3 and substrate during histone H2A ubiquitination by RNF168. H2A is one of the histone proteins composing the nucleosome core. H2A is abundantly modified on its C-terminal tail at K119 by the RING E3 ligases present in the Polycomb repressive complex 1 (PRC1), where RING1B/BMI1 is the most studied E3 dimer [12] , [13] , [31] , [32] . Recently, the E3 ligase RNF168 has been described to target the N-terminal residues K13–15 during DNA double-strand break signalling [14] , [15] . RNF168 is a monomeric E3 ligase that is recruited to sites of DNA damage by interaction of its conserved ubiquitin interaction motives with ubiquitin chains [33] , [34] , [35] , [36] , [37] . Its recruitment depends on the signalling of a large number of other proteins that are localized at damage sites with faster kinetics [35] , [36] , [37] . Once RNF168 is localized at these sites, its ability to target K13–15 on H2A is required for a functional response cascade [14] , [20] , [38] . This ubiquitination reaction is highly selective for K13–15 in cells and interestingly the RING domain of the E3 is sufficient to confer target specificity in vitro with the E2 UbcH5c [14] , [20] . This provides a useful system for mechanistic studies of the molecular determinants on the E3 and the substrate that regulate this specificity. In this study we identify the region on the RING domain of RNF168 that interacts with its targets, namely the nucleosomes and H2A/H2B dimers. We find that these substrates activate the RNF168-dependent reaction and this effect is dependent on a conserved acidic patch present on the H2A/H2B surface. These findings indicate that RNF168-dependent K13–15 modification is regulated by a region located distally to the target lysines. In addition, they highlight the importance of accessibility to the acidic patch by the ubiquitination machinery during DNA damage signalling. RNF168 can site-specifically modify H2A/H2B dimers We previously showed that the E3 ligase RNF168 is specific for K13 and K15 on H2A in oligonucleosomes in vivo and in vitro [14] . Here by using recombinant nucleosome core particles (NCPs) carrying lysine mutations on H2A we find that, although eventually other lysines are also modified, the RING domain of RNF168 is sufficient to favour modification of the K13–15 lysines in vitro ( Supplementary Fig. 1a ). As we use a RNF168 construct (R; residues 1–189), carrying not only the RING domain but also the MIU1 and UMI motives [33] , [34] , [35] , [36] , [37] we wondered if specificity for the K13–15 site is affected upon deletion of these ubiquitin-binding regions ( Supplementary Fig. 1b ). With a minimal RING domain construct (residues 1–113) we observe a decrease in activity towards H2A in NCPs but the specificity for K13–15 is retained ( Supplementary Fig. 1c ), confirming that the short RING domain provides the observed lysine specificity [20] . Next, we investigated the minimal substrate requirements for RNF168 activity. As previously shown [14] , RNF168 can target the isolated histone H2A in vitro in an aspecific manner, as the K13–15R mutant is modified at similarly low levels as WT H2A ( Fig. 1a ). This is not surprising as the histone in isolation is mostly unfolded. 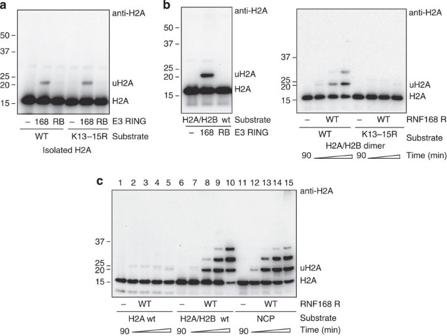Figure 1: The H2A/H2B dimer is specifically modified at K13–15 by the RNF168 RING domain. (a) RNF168 targets H2A in isolation in an inefficient manner and its activity is not specific for K13–15. RING1B/BMI1 are inactive towards the histone protein alone. Ubiquitination assay performed in presence of H2A WT or K13–15R in isolation. (b) RNF168 targets H2A specifically on K13–15 within the H2A/H2B dimer. Ubiquitination assays performed in presence of WT or K13–15R H2A in H2A/H2B dimer. Single time-point assay, where RING1B/BMI1 were used as negative control. Time course assay (10–30–60–90 min) in the presence of WT or K13–15 R dimers (assays performed at 200 mM NaCl). (c) RNF168 has comparable activity for H2A in dimers and in nucleosomes, while isolated H2A is targeted with low efficiency. Time course assay (10–30–60–90 min) to compare activity of RNF168 RING domain towards H2A alone, H2A/H2B dimers and NCPs. Figure 1: The H2A/H2B dimer is specifically modified at K13–15 by the RNF168 RING domain. ( a ) RNF168 targets H2A in isolation in an inefficient manner and its activity is not specific for K13–15. RING1B/BMI1 are inactive towards the histone protein alone. Ubiquitination assay performed in presence of H2A WT or K13–15R in isolation. ( b ) RNF168 targets H2A specifically on K13–15 within the H2A/H2B dimer. Ubiquitination assays performed in presence of WT or K13–15R H2A in H2A/H2B dimer. Single time-point assay, where RING1B/BMI1 were used as negative control. Time course assay (10–30–60–90 min) in the presence of WT or K13–15 R dimers (assays performed at 200 mM NaCl). ( c ) RNF168 has comparable activity for H2A in dimers and in nucleosomes, while isolated H2A is targeted with low efficiency. Time course assay (10–30–60–90 min) to compare activity of RNF168 RING domain towards H2A alone, H2A/H2B dimers and NCPs. Full size image In contrast, when a reconstituted dimer of H2A and H2B is provided as substrate, the RING domain of RNF168 can modify the WT protein efficiently, but not the K13–15R variant, indicating that the reaction becomes specific for these lysines on H2A ( Fig. 1b ). These findings indicate that the isolated H2A/H2B dimer is sufficient to provide H2A lysine specificity for the RNF168 RING domain reaction. When we compare the activity of RNF168 towards H2A, the H2A/H2B dimer and NCPs, we observe that rates of modification for dimer and NCP are very similar and much higher than on H2A alone ( Fig. 1c ), showing that the histone dimer contains the minimal molecular features that define the relevant substrate for RNF168 activity. RNF168 RING uses a charged region for nucleosome recognition To understand how the RNF168 RING domain recognizes its substrate, we first set out to identify the region on the RING domain involved in nucleosome interactions. We have previously shown that a charged residue located adjacent to the second Zn ion in the RNF168 RING domain (R57, Fig. 2a ) is important for nucleosomal H2A ubiquitination but not for targeting the isolated histone or making ubiquitin chains [14] . 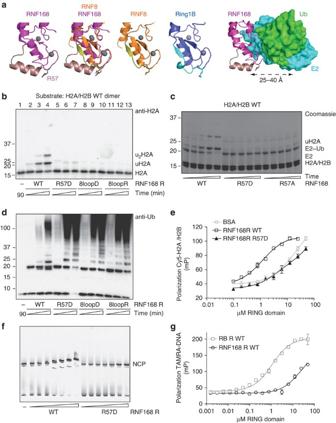Figure 2: RNF168 RING domain interacts with the target through a charged region. (a) Position of the targeting region on the RNF168 RING domain: 8loopD: replacement of residues 57–72 on RNF168 (PDB-code:3L11 (ref.54), in magenta) with residues 443–449 of RNF8 (PDB-code: 4AYC14, in orange). 8loopR: replacement of residues 58–72 on RNF168 with residues 444–449 of RNF8: R57 is present in this RING domain mutant. The residues in RNF8 used in the 8loopD mutant are highlighted in olivegreen (D443 in sticks). Position of the targeting region relative to E2 binding (model based on the RNF4/UbcH5a–Ub structure PDB-code: 4AP4 (ref.27)) (b) H2A/H2B dimer targeting by RNF168 requires both the helix (58–72) and R57. Anti-H2A blots of time course experiment (30–60–90 min) performed in the presence of H2A/H2B WT dimer (5 μM) and different mutants of RNF168 RING domain (1 μM). Anti-ubiquitin blot of these samples are shown ind. (c) Mutation of R57 to A or D inhibits the activity of the RING domain towards H2A/H2B dimers. Time course single turnover assay (1, 2, 4, 8 and 16 min), coomassie staining of SDS–PAGE gel. Appearance of ubiquitinated H2A is visible only in the presence of WT RNF168. Experimental conditions as inFig. 5b,c(100 nM E3). E2–Ub discharge occurs only in the presence of a targetable substrate. (d) Mutation of the helix (58–72) and R57 do not inhibit ubiquitin chain formation by RNF168 RING domain. Anti-ubiquitin blot of the samples shown inb. (e) RNF168 RING domain interacts with H2A/H2B dimers via the R57 site. FP assay usingCy-5H2A/H2B dimers (10 nM) and increasing amounts of RNF168 RING domain WT or R57D mutant. BSA is shown as a control to assess the effect of protein crowding in the reactions. Mean and s.e.m. are shown, calculated on at least two independent experiments. (f) RNF168 RING domain interacts with NCPs via the R57 site. Gel-shift assay performed in the presence of WT NCPs (100 nM) and increasing concentrations of RNF168 RING domain WT or R57D (0.77–1.55–3.1–6.2–12.5–25–50 μM). (g) RNF168 RING domain binds DNA with very low affinity at 50 mM NaCl, compared with the RING domains of RING1B/BMI1 (RB R). DNA binding measured by FP assay of TAMRA-labelled 15mer DNA. Mean and s.e.m. are shown, calculated on two replicates. Figure 2: RNF168 RING domain interacts with the target through a charged region. ( a ) Position of the targeting region on the RNF168 RING domain: 8loopD: replacement of residues 57–72 on RNF168 (PDB-code:3L11 (ref. 54 ), in magenta) with residues 443–449 of RNF8 (PDB-code: 4AYC [14] , in orange). 8loopR: replacement of residues 58–72 on RNF168 with residues 444–449 of RNF8: R57 is present in this RING domain mutant. The residues in RNF8 used in the 8loopD mutant are highlighted in olivegreen (D443 in sticks). Position of the targeting region relative to E2 binding (model based on the RNF4/UbcH5a–Ub structure PDB-code: 4AP4 (ref. 27 )) ( b ) H2A/H2B dimer targeting by RNF168 requires both the helix (58–72) and R57. Anti-H2A blots of time course experiment (30–60–90 min) performed in the presence of H2A/H2B WT dimer (5 μM) and different mutants of RNF168 RING domain (1 μM). Anti-ubiquitin blot of these samples are shown in d . ( c ) Mutation of R57 to A or D inhibits the activity of the RING domain towards H2A/H2B dimers. Time course single turnover assay (1, 2, 4, 8 and 16 min), coomassie staining of SDS–PAGE gel. Appearance of ubiquitinated H2A is visible only in the presence of WT RNF168. Experimental conditions as in Fig. 5b,c (100 nM E3). E2–Ub discharge occurs only in the presence of a targetable substrate. ( d ) Mutation of the helix (58–72) and R57 do not inhibit ubiquitin chain formation by RNF168 RING domain. Anti-ubiquitin blot of the samples shown in b . ( e ) RNF168 RING domain interacts with H2A/H2B dimers via the R57 site. FP assay using Cy-5 H2A/H2B dimers (10 nM) and increasing amounts of RNF168 RING domain WT or R57D mutant. BSA is shown as a control to assess the effect of protein crowding in the reactions. Mean and s.e.m. are shown, calculated on at least two independent experiments. ( f ) RNF168 RING domain interacts with NCPs via the R57 site. Gel-shift assay performed in the presence of WT NCPs (100 nM) and increasing concentrations of RNF168 RING domain WT or R57D (0.77–1.55–3.1–6.2–12.5–25–50 μM). ( g ) RNF168 RING domain binds DNA with very low affinity at 50 mM NaCl, compared with the RING domains of RING1B/BMI1 (RB R). DNA binding measured by FP assay of TAMRA-labelled 15mer DNA. Mean and s.e.m. are shown, calculated on two replicates. Full size image First, we observed that the R57D RING domain mutant has lost activity towards H2A in the H2A/H2B dimer ( Fig. 2b ), indicating that the function of this residue is retained when only H2A and H2B are present. Additionally, we tested an RNF168 R57A mutant RING domain. This protein also inhibits the E3 ligase function towards the histone dimer ( Fig. 2c ), excluding the possibility that the observed effect is caused by electrostatic repulsion of the aspartate mutant. To further explore this region on the RING domain we analysed the importance of a helix adjacent to this site in RNF168, rich in positively charged residues. We replaced this helix (residue 58–72, Fig. 2a ) with a shorter loop that is present on RNF8, an E3 ligase that is inactive towards nucleosomal H2A [14] (residues 444–449, Fig. 2a ). The constructs include either the helix alone (8loopR) or the helix and the R57D mutation (8loopD). Neither of these mutants is affected in its ability to promote ubiquitin chain formation ( Fig. 2d ). Nevertheless, both of these have lost the ability to modify H2A within the H2A/H2B dimer ( Fig. 2b ). Overall, these results show that both R57 and the adjacent helical region on the RING domain of RNF168 are required for H2A modification. To test whether this region is involved in direct interaction with the substrate, we analysed binding of the RNF168 RING domain to recombinant NCPs using native gel-shift assays and to H2A/H2B dimers using fluorescence polarization (FP) experiments. The RING domain of RNF168 binds to H2A/H2B dimers with an apparent dissociation constant (Kd) of ~1 μM ( Fig. 2e ) and it can shift NCPs on a native gel ( Fig. 2f ). In contrast, the R57D mutant shows impaired binding to both substrates ( Fig. 2e,f ), indicating a role for this site in direct interaction with the H2A/H2B dimer and the NCPs. In the RING domain of RING1B ( Fig. 2a ), the structurally analogous region to this C-terminal helix is involved in DNA binding and thereby in target recognition [25] , therefore we tested the DNA binding capacity of the RING domain of RNF168. In a buffer containing 50 mM NaCl, RING1B/BMI1 binds a double-strand 15mer DNA (Kd~1–1.5 μM, Fig. 2g ) [25] . In contrast, even at this low salt concentration, RNF168 shows very weak interaction with DNA (>10 μM, Fig. 2g ). At higher salt concentrations no binding is observed. This indicates that RNF168 doesn’t recognize NCPs through DNA interactions, in line with the observation that the H2A/H2B dimer is sufficient to provide an efficient substrate. Overall, these data show that RNF168 RING domain binds the H2A/H2B dimer and the nucleosomes. The charged region at the C-terminal end of the RING domain of RNF168 is involved in this binding and thereby in substrate selection. Mutations in this positively charged region impair the RNF168-mediated H2A modification by disrupting the binding to its substrate, the NCPs. Notably, the intrinsic free ubiquitin chain forming activity of RNF168 is not affected in these mutants ( Fig. 2d ). H2A modification requires an intact nucleosomal acidic patch We next investigated how the H2A/H2B dimer confers selectivity to the RNF168-driven reaction. The H2A/H2B dimer is known to form an acidic patch on the surface of the nucleosome core, by clustering several glutamate residues from H2A and H2B ( Fig. 3a ). This acidic patch is employed by a variety of proteins, including the H4 tail, for binding to the nucleosomes in different processes [38] . To investigate a potential role for this patch in the RNF168 reaction, we assembled H2A/H2B dimers with mutant histones (E61,64,91A on H2A and/or E102,110A on H2B). These mutations do not affect the formation of the H2A/H2B dimers ( Supplementary Fig. 2a ), but they prevent RNF168-dependent H2A ubiquitination ( Fig. 3b ). Similar results were obtained when we reconstituted NCPs with all five glutamates mutated (NCP EA) indicating that the integrity of this patch is required for productive ubiquitination by RNF168 ( Fig. 3c ). 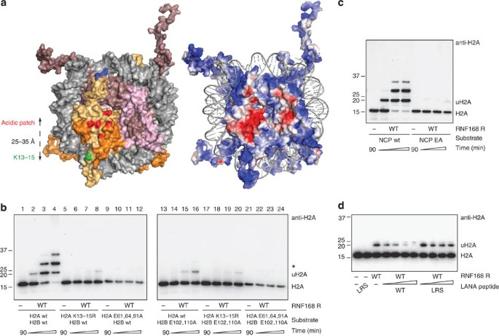Figure 3: Targeting H2A requires an intact and accessible acidic patch. (a) Position of the acidic patch within the nucleosome. NCP structure (1KX5 (ref.55)) where H2B is shown in orange, H2A in yellow–orange, H3 in light pink and H4 in violet. K118–119 on H2A are highlighted in blue, K13–15 are in green and the glutamate residues of the acidic patch are shown in red. Distance between K13–15 and the acidic patch are indicated on the left. Electrostatic potential (red is negative, blue is positive) of the histone core in the NCP highlights the acidic patch on the surface of the H2A/H2B dimer. (b) Mutations in the acidic patch on H2A or H2B impair H2A ubiquitination in H2A/H2B dimers. Time course experiment (30–60–90 min) following activity of RNF168 RING domain towards H2A in the different H2A/H2B mutant dimers. (c) Acidic patch mutations prevent ubiquitination of NCPs. Time course experiment (30–60–90 min) to investigate the activity of RNF168 RING domains towards H2A in nucleosome WT or EA (H2A E61, 64, 91 Å and H2B E102, 110 Å). (d) Binding of a LANA peptide, but not a mutant LRS variant, to the nucleosome competes with RNF168-dependent ubiquitination of NCPs. Ubiquitination assay with 3–10–30–100 μM peptide. Note that E91 on H2A is part of the epitope recognized by the anti-H2A antibodies; therefore, there is reduced signal on western blots when the E91A mutation is introduced. Figure 3: Targeting H2A requires an intact and accessible acidic patch. ( a ) Position of the acidic patch within the nucleosome. NCP structure (1KX5 (ref. 55 )) where H2B is shown in orange, H2A in yellow–orange, H3 in light pink and H4 in violet. K118–119 on H2A are highlighted in blue, K13–15 are in green and the glutamate residues of the acidic patch are shown in red. Distance between K13–15 and the acidic patch are indicated on the left. Electrostatic potential (red is negative, blue is positive) of the histone core in the NCP highlights the acidic patch on the surface of the H2A/H2B dimer. ( b ) Mutations in the acidic patch on H2A or H2B impair H2A ubiquitination in H2A/H2B dimers. Time course experiment (30–60–90 min) following activity of RNF168 RING domain towards H2A in the different H2A/H2B mutant dimers. ( c ) Acidic patch mutations prevent ubiquitination of NCPs. Time course experiment (30–60–90 min) to investigate the activity of RNF168 RING domains towards H2A in nucleosome WT or EA (H2A E61, 64, 91 Å and H2B E102, 110 Å). ( d ) Binding of a LANA peptide, but not a mutant LRS variant, to the nucleosome competes with RNF168-dependent ubiquitination of NCPs. Ubiquitination assay with 3–10–30–100 μM peptide. Note that E91 on H2A is part of the epitope recognized by the anti-H2A antibodies; therefore, there is reduced signal on western blots when the E91A mutation is introduced. Full size image To confirm these findings, we performed ubiquitination assays using wild-type NCPs in presence of a peptide known to bind on the acidic patch (LANA) [39] . In these experiments, increasing amounts of LANA peptide were found to inhibit the ubiquitination of nucleosomal H2A. Using a mutant variant of this peptide (LRS), unable to bind the nucleosome [39] , did not affect the reaction ( Fig. 3d ). This supports the hypothesis that the acidic patch on the nucleosome is required for activity of the RNF168/UbcH5c ubiquitination machinery. The acidic patch is not involved in binding by RNF168/UbcH5c To analyse the importance of the acidic patch for recruitment of the E3, we compared binding of the RNF168 RING domain to wild-type or EA mutant NCPs and H2A/H2B dimers. Surprisingly, the presence or absence of the acidic patch does not affect the binding of RNF168 RING domain to these substrates ( Fig. 4a,b ). Moreover, binding of the RNF168 RING domain on wild-type NCPs cannot be competed out by the LANA peptide ( Fig. 4c ) although this does inhibit ubiquitination activity ( Fig. 3d ). 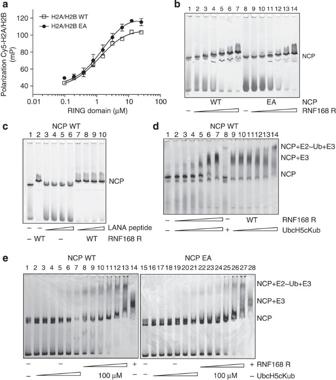Figure 4: The nucleosome interacts with the E2~Ub/E3 complex independently of the acidic patch. (a) Mutation of the acidic patch on H2A/H2B dimers does not affect RNF168 RING domain binding. FP assay using Cy-5-labelled H2A/H2B dimers (10 nM) and increasing amounts of RNF168 RING domain WT. Mean and s.e.m. are shown, calculated on at least two independent experiments. (b) The RNF168 RING domain binds equally well to NCPs with (WT) and without acidic patch (EA). Gel-shift assay with NCPs WT and EA (100 nM) and RNF168 RING domain (1.55–3.1–6.2–12.5–25–50 μM). (c) Binding to NCPs does not rely on the accessibility of the acidic patch. Gel-shift assay where NCPs WT (100 nM) are assessed for binding by RNF168 RING domain (25 μM) with increasing concentration of LANA peptide WT (12–25–50–100 μM). (d) The E2~Ub thioester shifts the E3–NCP complex at high concentrations. Gel-shift assay where WT NCPs (100 nM) are assessed for binding by RNF168 RING domain (3.1–6.2–12.5–25–50–100 μM, lanes 2–7) and/or UbcH5c~Ub (3.1–6.2–12.5–25–50–100 μM, lanes 9–14). In lanes 9–14 the E3 concentration was kept constant to 100 μM. (e) Both WT and EA NCPs can form an E2~Ub/E3/target complex. Gel-shift assay where NCPs WT (100 μM, lane 1–14) and EA (100 nM, lane 15–28) are assessed for binding by UbcH5c~Ub (3.1–6.2–12.5–25–50–100 μM, lanes 2–7/15–21) or for binding of RNF168 RING domain (3.1–6.2–12.5–25–50–100 μM, lane 8–13/22–27) in the presence of 100 μM UbcH5c~Ub. Figure 4: The nucleosome interacts with the E2~Ub/E3 complex independently of the acidic patch. ( a ) Mutation of the acidic patch on H2A/H2B dimers does not affect RNF168 RING domain binding. FP assay using Cy-5-labelled H2A/H2B dimers (10 nM) and increasing amounts of RNF168 RING domain WT. Mean and s.e.m. are shown, calculated on at least two independent experiments. ( b ) The RNF168 RING domain binds equally well to NCPs with (WT) and without acidic patch (EA). Gel-shift assay with NCPs WT and EA (100 nM) and RNF168 RING domain (1.55–3.1–6.2–12.5–25–50 μM). ( c ) Binding to NCPs does not rely on the accessibility of the acidic patch. Gel-shift assay where NCPs WT (100 nM) are assessed for binding by RNF168 RING domain (25 μM) with increasing concentration of LANA peptide WT (12–25–50–100 μM). ( d ) The E2~Ub thioester shifts the E3–NCP complex at high concentrations. Gel-shift assay where WT NCPs (100 nM) are assessed for binding by RNF168 RING domain (3.1–6.2–12.5–25–50–100 μM, lanes 2–7) and/or UbcH5c~Ub (3.1–6.2–12.5–25–50–100 μM, lanes 9–14). In lanes 9–14 the E3 concentration was kept constant to 100 μM. ( e ) Both WT and EA NCPs can form an E2~Ub/E3/target complex. Gel-shift assay where NCPs WT (100 μM, lane 1–14) and EA (100 nM, lane 15–28) are assessed for binding by UbcH5c~Ub (3.1–6.2–12.5–25–50–100 μM, lanes 2–7/15–21) or for binding of RNF168 RING domain (3.1–6.2–12.5–25–50–100 μM, lane 8–13/22–27) in the presence of 100 μM UbcH5c~Ub. Full size image These observations indicate that, in contrast to the RNF168 R57 site, the acidic patch on the target is not involved in the direct interaction with the E3 ligase. Since simple recruitment of the E3 ligase to the substrate does not explain the importance of the acidic patch for RNF168 activity, a different step in the ubiquitination reaction must be affected. We wondered whether the acidic patch would affect the formation of the NCP-E3-E2~Ub complex. We used a mutant UbcH5c where the active site cysteine is mutated to lysine (C85K) to form a stable isopeptide linkage with the C-terminal tail of ubiquitin [27] , preventing the release of the ubiquitin in presence of the E3 and the substrate. With this stable E2~Ub complex we could assess how the RING/E2~Ub complex binds to NCPs in gel-shift assays. In these assays the E2~Ub complex alone does not bind to NCPs ( Fig. 4d , lane 8 and 4e, lanes 1–6) but it causes an additional shift of the E3-NCP complex when E2~Ub is present at high concentrations (>25 μM) ( Fig. 4d ). This shows that a trimeric complex can assemble on NCPs containing E3/E2~Ub, although the E2~Ub component does not significantly alter the affinity of the RING for NCPs. Interestingly the trimeric complex is observed for both WT and EA NCPs with the charged E2 complex ( Fig. 4e ). This implies that its assembly takes place independently of the integrity of the acidic patch. We conclude that binding of the ubiquitination machinery to the substrate does not rely on the nucleosomal acidic patch. The acidic patch is critical for H2A ubiquitination by RNF168 Since the importance of the acidic patch for activity ( Fig. 3 ) is not explained by a role in binding ( Fig. 4 ), we postulated that these negative charges on the nucleosome core may have a role in the actual catalysis by the RNF168 RING domain and the E2 UbcH5c. To address this point we performed single turnover assays following the rate of ubiquitin discharge from UbcH5c in presence of RNF168 and of the different substrates. In these reactions, when the E3 concentration is low (100 nM), RNF168 is hardly capable to activate ubiquitin discharge ( Fig. 5a , lanes 4–5–6), compared to conditions where we use 1 μM E3 concentrations ( Fig. 5a , lanes 10–11–12). Nevertheless, when substrate (NCPs) was added to the reactions, we observed a drastic activation of the discharge rate even at these low RNF168 concentrations ( Fig. 5a , lanes 1–2–3). This effect was not observed in absence of RNF168 ( Fig. 5a , lanes 13–14–15), confirming that the NCPs alone do not promote discharge of the E2~Ub complex. 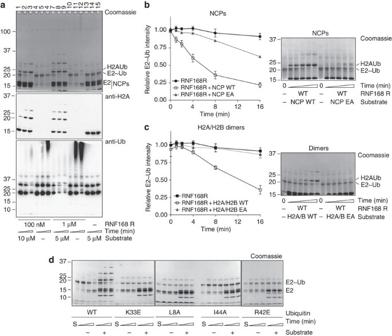Figure 5: The active role of the substrate in the reaction depends on the acidic patch. (a) The substrate activates the discharge of ubiquitin from the E2 by RNF168 RING domain. Single turnover experiment performed at different E3 concentration shows that in the presence of NCPs, there is activation of the enzymatic activity of RNF168 RING domain. The NCPs alone, in absence of RNF168, (lanes 13–15) are unable to stimulate E2 discharge. (b,c) NCPs (b) and H2A/H2B dimers (c) further stimulate E2 discharge by RNF168. In the absence of the charges on the acidic patch the substrate-dependent activation is not taking place. Quantification of time course single turnover assays (1, 2, 4, 8 and 16 min), where peak height of the E2~Ub band was used from Coomassie-stained SDS–PAGE gels. Example gels are shown; the gels were run for longer time to increase the separation between the E2~Ub and the H2Aub bands. The samples at time 0 were used for the normalization. At least two independent experiments per time point and condition where used for quantification. Mean and s.e.m. are shown. E3 (100 nM) was used in these reactions. (d) Ubiquitin residues required for E3 allosteric activation are important in the reaction towards the substrate. Single turnover assays in presence and absence of NCPs performed with 20 μM E2~Ub and 1 μM E3 and 5 μM substrate, time course 1.5–3–4–6–8 min. The R42E ubiquitin mutant samples were run using oligonucleosomes and not recombinant NCPs. Figure 5: The active role of the substrate in the reaction depends on the acidic patch. ( a ) The substrate activates the discharge of ubiquitin from the E2 by RNF168 RING domain. Single turnover experiment performed at different E3 concentration shows that in the presence of NCPs, there is activation of the enzymatic activity of RNF168 RING domain. The NCPs alone, in absence of RNF168, (lanes 13–15) are unable to stimulate E2 discharge. ( b , c ) NCPs ( b ) and H2A/H2B dimers ( c ) further stimulate E2 discharge by RNF168. In the absence of the charges on the acidic patch the substrate-dependent activation is not taking place. Quantification of time course single turnover assays (1, 2, 4, 8 and 16 min), where peak height of the E2~Ub band was used from Coomassie-stained SDS–PAGE gels. Example gels are shown; the gels were run for longer time to increase the separation between the E2~Ub and the H2Aub bands. The samples at time 0 were used for the normalization. At least two independent experiments per time point and condition where used for quantification. Mean and s.e.m. are shown. E3 (100 nM) was used in these reactions. ( d ) Ubiquitin residues required for E3 allosteric activation are important in the reaction towards the substrate. Single turnover assays in presence and absence of NCPs performed with 20 μM E2~Ub and 1 μM E3 and 5 μM substrate, time course 1.5–3–4–6–8 min. The R42E ubiquitin mutant samples were run using oligonucleosomes and not recombinant NCPs. Full size image As quantified in Fig. 5b,c , the activating contribution of the substrate to the RNF168 reaction was observed both for NCPs and H2A/H2B dimers ( Fig. 5b,c , open boxes). Moreover, in these experiments we also noticed that the substrate seems to redirect the ubiquitination from chain formation to target protein modification. While the sole addition of the RNF168 RING domain increases the amount of ubiquitin conjugates in the reaction as expected ( Fig. 5a , lanes 4–5–6–10–11–12 and Supplementary Fig. 3a,b , lanes 7–11), the concomitant addition of the substrate NCP or H2A/H2B dimer strongly reduces the formation of high molecular weight ubiquitin species in favour of H2A modification ( Fig. 5a , lanes 1–2–3–7–8–9 and Supplementary Fig. 3a , lanes 12–16 and 3b, lanes 13–17). This suggests that the substrate is actively involved in catalysis by directing the E2/E3 activity towards the target lysine on H2A. Interestingly, when we used NCPs or H2A/H2B dimers with mutation of the acidic patch (EA), the activation of the E2~Ub discharge due to the presence of the substrate was lost ( Fig. 5b,c , grey triangles) and the high-molecular weight ubiquitin chains were formed in similar amounts compared with the reactions where the substrate is not present ( Supplementary Fig. 3a , lanes 17–21 and 3b, lanes 18–22). These findings show that the acidic patch residues are critical for catalysis by RNF168/UbcH5c, without being involved in the interaction between the ubiquitination machinery and the target ( Fig. 4 ). In previous studies of the RING E3 mechanism it became clear that an important step in the reaction can be the positioning of ubiquitin for catalysis [26] , [27] , [28] , [29] , [30] . A possible function of the substrate in these reactions may cause a different catalytic mechanism by forcing a different orientation of ubiquitin in respect to the E3/E2 machinery to enhance the ubiquitin transfer. We investigated whether mutation of key residues critical in RING-dependent stabilization of an E2~ubiquitin complex [26] , [27] , [28] could affect the RNF168 reactions in presence or absence of the target. In these assays the I44, L8, R42 and K33 sites are required for both substrate-independent and -dependent reactions ( Fig. 5d ), indicating that RNF168-dependent catalysis is likely to utilize a similar mechanism as previously described [26] , [27] , [28] both in presence and in absence of the substrate. This suggests that the acidic patch effect during the RNF168 reaction is not due to a repositioning of the ubiquitin moiety in the ubiquitination complex. Moreover, since mutation of the residues forming the acidic patch on either H2A or H2B individually has comparable effects ( Fig. 3a ), it seems likely that the role of the acidic patch is not mediated by a single glutamate residue involved in catalysis, but rather that the nucleosomal negative surface at this region influences the reaction by RNF168/UbcH5c, either by orienting the machinery or by long-range effects on the catalysis ( Fig. 6a ). 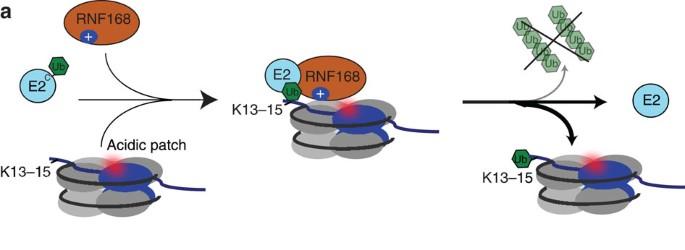Figure 6: The nucleosomal acidic patch is critical for RNF168 reaction. (a) The ubiquitination of K13–15 on H2A in nucleosomes requires a positive patch on RNF168 for the recruitment of the E3 ligase to the H2A/H2B dimer and the nucleosome. The negatively charged acidic patch formed by H2A and H2B activates and redirects the reaction from chain formation to selective H2A modification. Figure 6: The nucleosomal acidic patch is critical for RNF168 reaction. ( a ) The ubiquitination of K13–15 on H2A in nucleosomes requires a positive patch on RNF168 for the recruitment of the E3 ligase to the H2A/H2B dimer and the nucleosome. The negatively charged acidic patch formed by H2A and H2B activates and redirects the reaction from chain formation to selective H2A modification. Full size image The mechanism of RING-dependent ubiquitination reactions is complex and does not involve enzymes with conventional catalytic properties. Recent studies have highlighted how RING domains allosterically activate the release of ubiquitin from the E2 (refs 26 , 27 , 28 ), but relatively little is known about the influence of the substrate on the reaction. H2A ubiquitination is particularly interesting because the RING domains of the respective E3 ligases can provide lysine specificity to the in vitro reactions with the same E2 enzyme, UbcH5c. Therefore, the RING domains of PRC1 and RNF168 must contain the molecular requirements to orient themselves, providing a minimal system for studying substrate recognition and its role in the catalytic process. This study focuses on the recently described K13–15 ubiquitination of H2A by RNF168, which has roles in the DNA damage signalling. We showed that the isolated H2A/H2B dimer is the minimal relevant substrate required for an efficient and specific reaction. Then, we identified a region on the RING domain of the E3 involved in substrate binding. Next, we found that the substrate is able to accelerate the reaction catalysed by RNF168/UbcH5c, redirecting ubiquitination activity towards the physiologically relevant lysines on H2A. These effects are highly dependent on an intact acidic patch on the H2A/H2B dimer within the nucleosome. The actual mechanism used by these substrates to regulate catalysis and the selectivity for specific lysines require further analysis. Particularly, the target lysines (K13–15) are likely to play a role in this mechanism, but we have not succeeded in uncoupling the contribution of these residues, because the lysine mutants are still modified in these in vitro reactions. Nevertheless, our results are important for understanding the mechanistic aspects of the RNF168 reaction as well as its functional requirements in the biological context of DNA damage signalling. The acidic patch is located far from the target lysine, providing the first distal substrate region with a direct role in ubiquitination catalysis beyond mere binding. This proposes a novel role for substrates in ubiquitination reactions that may well be more general, although it is unlikely that all ubiquitination targets will contribute to ubiquitination reactions in this manner. When the target is non-specific and it is not important which lysine is modified, as proposed for example for Cullin-mediated reactions [40] , such an involvement is less likely. For cases where the lysine location is a critical signal, however, the catalytic involvement of the substrate can provide an important step in optimizing selectivity and efficiency of the ubiquitination reaction, with unique aspects. Such a complex mechanism ensures that modification takes place only when sufficient E3/E2~Ub is available that contacts the substrate in a specific configuration, where two conditions are met: the lysine is available in proximity to the E2~ubiquitin thioester and the machinery can cross-talk to a distal region involved in the activation. Active involvement of the substrate may explain the low-affinity interactions that are observed between RING E3s and their substrates, since it adds a regulatory step additional to proper target recognition. Our data show that RNF168 requires accessibility to the acidic patch on nucleosomes to target H2A. A large number of proteins are known to bind to this site, and RNF168 will have to compete with those to exert its function at DNA double-strand breaks sites. RNF168 is recruited to damaged chromatin by binding to ubiquitin chains, controlling the local concentration. The low affinity we measure for the E3 to the substrate ensures a dependence on the recruitment step and prevents premature action of RNF168. Here we propose that RNF168 reaction can only progress after adequate preparation of the chromatin fibres around the site of damage, where the acidic patch will be exposed. Many proteins are known to act upstream of RNF168, including E3 ligases such as RNF8 and HERC2 and other enzymes, for example, ATM and chromatin remodelers [35] , [36] , [37] , [41] , [42] , [43] , [44] , [45] , [46] . Some of these are required to recruit RNF168, but it is plausible that others are necessary to create the proper chromatin conformation around the damage that allow access to the acidic patch and hence promote ubiquitination of H2A. In addition, our study highlights that different histone H2A variants with alterations to the acidic patch residues may be treated differently by RNF168, for example, H2A.Bbd and H2A.Z [47] , [48] . Overall, our findings contribute to the understanding of the molecular requirements necessary for proper RNF168 activity on nucleosomal H2A and to the clarification of the necessary steps required for DNA damage signalling in response to DNA double-strand breaks. Protein expression and purification E1 was purified using His-tag affinity purification, PorosQ and gel-filtration columns [49] . UbcH5c was purified by GST-tag affinity purification and gel filtration after tag cleavage; untagged ubiquitin was purified by perchloric acid precipitation, Sepharose SP and Superdex 75 columns [13] , [14] . RNF168 (1–189) and RING1B/BMI1 RING domains were purified using a His-SUMO tag and a GST- and His-tags respectively, after cleavage of the tag, the proteins were run on a Superdex 75 column [13] , [14] . Oligonucleosomes were purified from HEK-293T cells [13] , [14] . Histone proteins were purified in denaturing conditions [50] . All point mutants, the RING loop substitutions and the acidic patch mutants were generated using the quickchange site-directed mutagenesis kit (Agilent Technologies). RNF168 (1–113) was cloned into a pGEX6p vector and it was expressed in E. coli with an overnight induction with 0.2 mM IPTG at 16 °C. After lysis in buffer containing 30 mM Hepes 8.0, 500 mM NaCl, 10% glycerol, 1 μM ZnCl 2 , 1 mM TCEP, the protein was purified using GSH beads (GE healthcare) and eluted with 50 mM glutathione. The tag was cleaved by GST-3c overnight in dialysis with lysis buffer. After removal of the protease, the uncleaved protein and the GST with GSH beads, the protein was loaded into a Superdex 75 column (GE healthcare) in 30 mM Hepes 8.0, 250 mM NaCl, 1 μM ZnCl 2 and 1 mM TCEP. The fractions containing the protein were concentrated and stored at −80 °C. SDS–PAGE of the final sample is shown in Supplementary Fig. 1b . Histone dimers were prepared by mixing H2A and H2B proteins in denaturing buffer. After refolding in dialysis tubes against 20 mM HEPES (pH 7.5), 2 M NaCl and 0.5 mM EDTA and 0.5 mM TCEP at 4 °C overnight, the dimer was purified by gel filtration on a S200 column (GE Healthcare) in 20 mM HEPES (pH 7.5), 2 M NaCl and 0.5 mM EDTA and 0.5 mM TCEP, then concentrated and stored at −80 °C. To minimize the NaCl contribution in the assays containing dimers, gel filtration in the presence of buffer containing 500 mM NaCl was performed. The elution profile of the dimers in this condition remained unaltered. Assays shown in Figs 3 and 5 were performed with dimers stored at 500 mM NaCl. NCPs were prepared using a KCl gradient (2–0.15 M) [51] , [52] . DNA used for the reconstitution was the 167 bp Widom 601 sequence [53] . The final purification step was a DEAE ion exchange column instead of preparative gel electrophoresis. After the linear salt gradient, NCPs were stored at 4 °C in 20 mM HEPES (pH 7.5), 200 mM KCl, 0.5 mM EDTA and 0.5 mM TCEP; for longer storage at −80 °C a final concentration of 20% glycerol was added to the samples. Mutant proteins were treated and prepared as wild type. In vitro ubiquitination assays All in vitro ubiquitination assays (except those involving discharge assays in Figs 2c and 5 and Supplementary Fig. 3 ) were performed as follows: E1 (0.2 μM) was mixed with UbcH5c (0.5 μM), E3 ligase (0.5–1 μM), ubiquitin (3–5 μM), ATP (3 mM) and 1 μM of histone H2A, H2A/H2B dimer or NCPs. The reactions were incubated at 32 °C for 90 min (unless otherwise stated) in buffer 50 mM Tris/HCl (pH 7.5), 100 mM NaCl, 10 mM MgCl 2 , 1 μM ZnCl 2 and 1 mM TCEP. Final salt concentration in the assays was normally ~150 mM, unless otherwise stated. Western blot analysis was performed using anti-H2A (Millipore 07–146, 1:1,000 dilution) or anti-ubiquitin (Santa Cruz P4D1, 1:1,000 dilution) antibodies, followed by secondary HRP-conjugated anti-rabbit or anti-mouse antibodies respectively (BioRad, 1:10,000 dilution). E2 discharge assays For the single turnover assays, the E2 was pre-charged with ubiquitin. Concentrations are given for Figs 2c and 5 , in brackets for Fig. 5 and Supplementary Fig. 3 . To load the E2, E1 at 0.5 μM was mixed with 100 μM (70 μM) UbcH5c in the presence of 100 μM (70 μM) ubiquitin Mg 2+ and 3 mM ATP in buffer, 50 mM Tris/HCl (pH 7.5), 100 mM NaCl and 10 mM MgCl 2 . The sample was incubated for 30–60 min at room temperature. The reaction was stopped with 50 mM EDTA final concentration and incubated on ice for 2 min. This mixture was then used for the discharge reactions, a final concentration of 15 μM (20 μM) E2~Ub was incubated at 32 °C with 100 nM (1 μM) of RNF168 RING domain alone or in the presence of 10 μM (5 μM) NCPs or 20 μM (5 μM) dimers. Samples were stopped at given times and were analysed by Coomassie staining on SDS–PAGE in non-reducing conditions and subsequently western blot analysis was carried out using anti-H2A (Millipore, 07–146) or anti-Ub (Santa Cruz, P4D1) antibodies. Samples were run on either 12% or 4–12% NuPAGE gels in MOPS buffer (Life Technologies). Images were taken using ChemiDoc XRS system (BioRad) and ImageLab programme. Quantifications were done using the peak height value of the E2~Ub band on Coomassie gels in ImageLab and GraphPad was used to prepare graphs. FP assay DNA-binding reactions were carried out with 5 nM TAMRA-labelled DNA (TAACCCTAACCCCTA), 25 mM HEPES (pH 7.4), 50 mM NaCl, 0.5% ( w / v ) BSA and 0.5% ( v / v ) Triton X-100. The RING domain protein solutions with the highest concentration were prepared in this buffer and subsequent dilutions were achieved by serial 1:1 dilutions in two repeats. The reaction was incubated for 15 min at room temperature before the measurements. For H2A/H2B dimer affinity studies an H2A mutant carrying an additional cysteine at the N terminus was engineered using PCR site-directed mutagenesis. The cysteine was labelled with a Cy-5 maleimide dye (GE Healthcare) using a 1:5 excess of dye over protein. The labelling reaction was carried out for 8 h at room temperature and stopped with 10 mM DTT. This mutant was used to prepare Cy-5 H2A/H2B dimers, following the same protocol used to prepare wild-type dimers. To assess binding of RNF168 to Cy-5 H2A/H2B dimer, 10 nM of labelled dimer was titrated with increasing concentrations of RNF168 RING domain in a buffer containing 50 mM Tris pH 7.5, 100 mM NaCl, 10 mM MgCl 2 1 mM TCEP and 0.05% TWEEN20. The reaction was incubated for 5 min at room temperature before the measurement. FP was measured in 384 low-volume plates (Corning) using a PHERAstar plate reader (BMG Labtech) with a FP filter module, with an excitation filter of 540 nm and an emission filter of 590 nm for TAMRA DNA and Ex 590 nm, Em 675 nm for Cy-5 H2A/H2B. The data were analysed with GraphPad and fitted to a one-site binding model ( Y = B max × X /( K d + X )+offset). UbcH5c C85K loading The C85K mutation was inserted in pGEX6p, UbcH5c; the protein was expressed in E. coli with an overnight induction at 16 °C with 0.2 mM IPTG. After lysis in buffer containing 50 mM Hepes (pH 8), 150 mM NaCl, 0.5 mM TCEP the protein was purified using GSH beads (GE Healthcare) and eluted with 50 mM glutathione. The tag was cleaved by GST-3c overnight in dialysis with lysis buffer. After removal of the protease, the uncleaved protein and the GST with GSH beads, the protein was loaded into a S75 column in 20 mM Hepes (pH 8.0), 150 mM NaCl and 1 mM TCEP. The fractions containing the protein were concentrated and stored at −80 °C. The mutant E2 was loaded in a reaction containing 200 μM UbcH5c C85K, 200 μM ubiquitin, 1 μM Uba1 and 50 mM Tris (pH 9.5), 150 mM NaCl, 0.8 mM TCEP, 3 mM ATP and 5 mM MgCl 2 (ref. 27 ). The reaction was incubated at 35 °C for ~20 h. The E2~Ub complex was purified on a S75 gel-filtration column and the fractions containing only the loaded E2 were concentrated and used for the gel-shift analysis shown in Fig. 4d,e . Gel-shift experiments Gel-shift assays were performed using native gel electrophoresis on 4–12% Pre-Cast Tris-Glycine gels (Life Technologies), pre-run for at least 1 h at 125 V in Novex Tris-Glycine buffer. NCPs (100 nM) were incubated with increasing amounts of E3 and/or E2~Ub in Shift Buffer (50 mM Tris (pH 7.5), 150 mM NaCl, 2 mM arginine, 0,01% CHAPS and 0.01% Nonidet P-40). Loading buffer (5 × ) containing 40% sucrose and 0.25% bromophenol blue was added to the sample and 5 μl of the samples were loaded and the gel was run for 90 min at 125 V. Gels were stained with GelRed and visualized using the ChemiDoc XRS and ImageLab. How to cite this article: Mattiroli, F. et al. The nucleosome acidic patch plays a critical role in RNF168-dependent ubiquitination of histone H2A. Nat. Commun. 5:3291 doi: 10.1038/ncomms4291 (2014).